Revealing composition and structure dependent deep-level defect in antimony trisulfide photovoltaics Antimony trisulfide (Sb 2 S 3 ) is a kind of emerging light-harvesting material with excellent stability and abundant elemental storage. Due to the quasi-one-dimensional symmetry, theoretical investigations have pointed out that there exist complicated defect properties. However, there is no experimental verification on the defect property. Here, we conduct optical deep-level transient spectroscopy to investigate defect properties in Sb 2 S 3 and show that there are maximum three kinds of deep-level defects observed, depending on the composition of Sb 2 S 3 . We also find that the Sb-interstitial (Sb i ) defect does not show critical influence on the carrier lifetime, indicating the high tolerance of the one-dimensional crystal structure where the space of (Sb 4 S 6 ) n ribbons is able to accommodate impurities to certain extent. This study provides basic understanding on the defect properties of quasi-one-dimensional materials and a guidance for the efficiency improvement of Sb 2 S 3 solar cells. Point defect engineering of semiconducting materials is essential for photovoltaic devices, comprehensive understanding of the defect formation mechanism and function enables achieving high-efficiency solar energy conversion. In specific, the point defect (intrinsic or extrinsic defect) determines the Fermi level ( E F ), free carrier concentration, and conductivity type (n or p) of semiconductors. Shallow-level defects with thermal energy of about k B T (where k B is Boltzmann constant, T is temperature) from conduction band minimum (CBM) or valence band maximum (VBM) play the major role to tune the carrier concentrations and conductivity type. In contrast, deep-level defect whose activation energy is much higher than k B T from CBM or VBM is detrimental to photogenerated carrier lifetime and transport (carrier mobility and diffusion length) [1] . These defects result in the trap-assisted Shockley–Read–Hall [2] , [3] (SRH) recombination (dominant non-radiation recombination) in solar cells, which is the primary cause of open-circuit voltage ( V OC ) loss. Recently, binary antimony chalcogenides Sb 2 S(e) 3 (including Sb 2 S 3 , Sb 2 Se 3 , Sb 2 (S, Se) 3 alloy) have drawn increasing attention in solar cell applications, for their large visible light absorption coefficient (>10 5 cm −1 ), earth-abundant compositional elements, and tunable band gap in 1.1–1.7 eV. The efficiency breakthrough towards 10% in alloy-type antimony selenosulfide stimulates new interests in the development of this class of materials [4] , [5] . In particular, Sb 2 S 3 with band gap of ~1.7 eV can be perfectly applied as top cell material for the construction of tandem solar cells. Different from previous photovoltaic materials such as silicon, Cu(In, Ga)Se 2 , CdTe, and organic–inorganic hybrid perovskite, the Sb 2 S 3 displays quasi-one-dimensional structure composed of [Sb 4 S 6 ] n ribbons and could generate benign grain boundaries without dangling bonds along c axis (Fig. 1 ) [6] , [7] . In practical, to transfer this distinctive structural advantage into efficient carrier transport and final power conversion efficiency (PCE), one must understand and control the defect properties, in particular the deep-level defects. This requirement has spurred intense interests in exploring the defect properties of such materials, especially from theoretical perspective, which revealed complicated defect characteristics although it has only two kinds of elements [8] , [9] , [10] , [11] . However, to date there is a lack of experimental verification of the defect properties associated with the structure and compositions, which induces ambiguity in the fabrication of high-quality Sb 2 S 3 films for efficient solar cells. Fig. 1: Schematic diagram of quasi-1-dimensional structural Sb 2 S 3 . Sideview ( a ) and aeroview ( b ) of [Sb 4 S 6 ] ribbons along c axis. Full size image Herein, we experimentally uncover the defect characteristics by using deep-level transient spectroscopy (DLTS) and identify the details of the defect. We examine both Sb-rich and S-rich Sb 2 S 3 films for a comparative study which are prepared by thermal evaporation approach. To make clear conclusions, we carefully analyze the crystallinity, electronic structure, and chemical composition (impurity) of the as-obtained films. In contrast to the theoretical study where complicated defect proposed in the Sb 2 S 3 [8] , [9] , [10] , [11] , our experimental investigation shows only a few types of defect, and the defect type and concentration are sensitively dependent on the anion/cation ratio. Structure and composition characterization of Sb 2 S 3 films Due to the high saturated vapor pressure of sulfur (50 mmHg at 300 °C) [12] , the sulfur loss is inevitable and results in Sb-rich Sb 2 S 3 films during the normal thermal evaporation deposition. To obtain S-rich Sb 2 S 3 film, we apply a co-evaporation equipment for the film fabrication, in which S powders are co-evaporated with Sb 2 S 3 for the generation of S-rich Sb 2 S 3 films. The synthesis details are provided in the Methods section. The as-obtained films at Sb-rich and S-rich conditions display similar morphology (Fig. 2a, b and Supplementary Fig. 1 ), featured as compact with clear grain boundaries. X-ray diffraction (XRD) is then applied to characterize the crystallinity (Fig. 2c ). Both of the films display diffractions at 15.6, 17.5, 24.9, 33.6, and 35.6°, which are well assigned as (020), (120), (130), (330), and (240) crystal planes of orthorhombic Sb 2 S 3 (JCPDS No. 42-1393, Pbnm ) [6] . 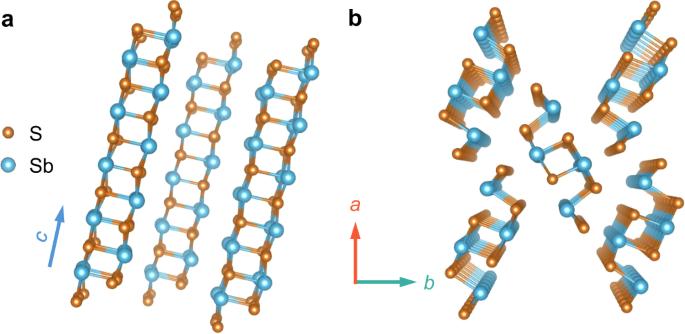Fig. 1: Schematic diagram of quasi-1-dimensional structural Sb2S3. Sideview (a) and aeroview (b) of [Sb4S6] ribbons alongcaxis. According to the energy dispersive X-ray spectroscopy (EDS), the atomic ratio of S/Sb in Sb-rich and S-rich Sb 2 S 3 films are calculated to be 1.28 to 1.55 (Supplementary Table 1 ), respectively. Fig. 2: Characterizations of Sb 2 S 3 films. a , b Surface SEM images of Sb-rich and S-rich Sb 2 S 3 films. c , d XRD patterns and Raman spectroscopy of Sb-rich and S-rich Sb 2 S 3 films. e , f Sb 3 d and S 2 p XPS spectra of Sb-rich and S-rich Sb 2 S 3 . Full size image Impurity crucially influences the defect properties in a semiconductor. In this case, we carry out Raman scattering and X-ray photoelectron spectroscopy (XPS) characterizations to carefully examine the bulk and surface chemical compositions. Raman spectra show typical asymmetric and symmetric bending vibration of S–Sb–S at 189 and 239 cm −1 (Fig. 2d ), respectively. The asymmetric and symmetric stretching vibration of Sb–S appear at 282 and 309 cm −1 . Furthermore, Raman shift at 126 and 156 cm −1 correspond to crystalline Sb 2 S 3 phase [13] . In addition, Raman shift at 302 cm −1 is ascribed to the phonon scattering from CdS substrate [14] . XPS spectra (Fig. 2e, f ) display typical binding energy of 539.2 eV and 529.8 eV which are assigned to Sb 3 d 3/2 and 3 d 5/2 of Sb 2 S 3 , respectively. Notably, there is no SbO x detected in both films, which is usually generated as impurity in the synthesis of Sb 2 S 3 and displays deep defect characteristics [15] . In addition, the binding energy of 163.1 eV and 161.9 eV are ascribed to the S 2 p 1/2 and 2 p 3/2 of Sb 2 S 3 [6] , [15] , [16] . In any case, from both Raman scattering and XPS analysis, both Sb-rich and S-rich Sb 2 S 3 films prepared via thermal evaporation are free of impurities, which thus provides excellent platform for the investigations of their defect properties. Photovoltaic performance of devices To test the optoelectronic quality of the as-synthesized film at device level, we examine the solar cell efficiency by using CdS and Spiro-OMeTAD as electron and hole transport layers (ETL & HTL), respectively (Fig. 3a, b ). The current density–voltage ( J–V ) curves are obtained under standard AM 1.5 G illumination (Fig. 3c ). The optimized Sb-rich Sb 2 S 3 film-based solar cell delivers PCE of 5.0%, with open-circuit voltage ( V OC ), short-circuit current density ( J SC ), and fill factor ( FF ) of 0.68 V, 15.4 mA cm −2 , and 47.6%, respectively. However, the optimized S-rich Sb 2 S 3 film-based device generates a PCE of 6.2% ( V OC of 0.72 V, J SC of 15.9 mA cm −2 , and FF 54.3%) with a net increase by 1.2% compared to the Sb-rich Sb 2 S 3 -based device. This PCE represents the highest value in thermal evaporation-derived Sb 2 S 3 solar cells [17] , [18] . The statistical parameters ( V OC , J SC , FF , and PCE) of each type of devices show narrow distributions (Supplementary Fig. 2a–e ), confirming the reliability of the film and device fabrication. Moreover, the external quantum efficiency (EQE) spectra (Fig. 3d and Supplementary Fig. 2f ) display excellent photocurrent generation efficiency in the 500–700 nm, a decrease in the short wavelength is attributed to the light absorption loss induced by CdS since its band gap is 2.4 eV. On the ground of both J–V and EQE analysis, the as-prepared S-rich Sb 2 S 3 films display high photovoltaic quality. Fig. 3: Device structure and photovoltaic performance. a , b Cross-sectional SEM image and corresponding device configuration of Sb 2 S 3 solar cells. c J–V characteristics of the optimal Sb-rich and S-rich Sb 2 S 3 devices under standard one Sun illumination. d EQE spectra of the optimized Sb-rich and S-rich Sb 2 S 3 -based devices. Full size image Bulk deep-level defects analysis We perform DLTS to gain insights into the defects in Sb 2 S 3 . In this characterization, there is a typical concern on the traditional electric DLTS regarding the distortion of minority-carrier trap detection [19] . However, attaching optical pulse to DLTS is recognized as an effective means to improve the sensitivity and authenticity of minority-carrier traps detection [20] , [21] . Herein, we adopt electric and optical double pulse mode, and both pulses are exerted simultaneously and share the same pulse width. In order to avoid the interference of ETL and HTL, a 635-nm wavelength red laser is selected as the source of optical pulse. Moreover, the reverse bias is set at −0.3 V, while various pulse voltages (0.1–0.5 V) are applied to avoid the fault peaks caused by the capacitance bridge recovery delay at inappropriate pulse voltage sometimes. Meanwhile, the defects at various depths can also be probed by varying the pulse voltage. Figure 4a, b shows the DLTS spectra of Sb-rich and S-rich Sb 2 S 3 devices at different pulse voltages. The positive peaks in the DLTS spectra represent majority-carrier traps, while the negative peaks indicate minority-carrier traps [19] . 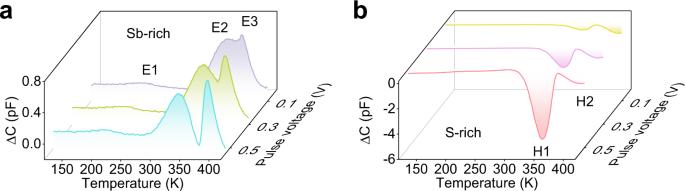Fig. 4: Deep-level defects characterization. DLTS signals of Sb-rich (a) and S-rich Sb2S3films (b) at pulse voltage ranging from 0.1 to 0.5 V, synergized with an identical pulse-width optical pulse. ΔCis the variation of capcitance. Regarding n-type Sb 2 S 3 (Supplementary note 1 ), the majority and minority-carrier traps are corresponding to electron and hole traps, respectively. Eventually, the statistical defects information of the two kinds of devices can be calculated and the results are summarized in Table 1 , where E T , σ , N T , τ , and N S are trap energy level, capture cross section, trap density, carrier lifetime, and shallow donor concentration (Supplementary note 2 ), respectively. It turns out that the Sb-rich film displays three electron traps, E1, E2, and E3 (donor defects), with the energy level of 0.31, 0.60, and 0.69 eV below the CBM (Figs. 4a and 5a ). In contrast, the S-rich film exhibits two hole traps which are denoted as H1 and H2 (acceptor defects) with energy levels of 0.64 and 0.71 eV above the VBM (Figs. 4b and 5b ). This characterization suggests clearly the composition-depended defect properties of Sb 2 S 3 films. Fig. 4: Deep-level defects characterization. DLTS signals of Sb-rich ( a ) and S-rich Sb 2 S 3 films ( b ) at pulse voltage ranging from 0.1 to 0.5 V, synergized with an identical pulse-width optical pulse. Δ C is the variation of capcitance. Full size image Table 1 Deep-level defect parameters (trap type, trap energy level ( E T ), capture cross section ( σ ), trap density ( N T ), carrier lifetime ( τ ), shallow donor concentration ( N S )) of Sb-rich and S-rich Sb 2 S 3 films. Full size table Fig. 5: Schematic of band structure and heterojunction. a , b Conduction band ( E C ), valence band ( E V ), Fermi level ( E F ), and trap energy level ( E T ) for Sb-rich and S-rich Sb 2 S 3 films. c Schematic diagram of V OC derived from split of electron and hole quasi Fermi level ( E Fn and E Fp ). Full size image According to the theoretical calculations [8] , [9] , the traps E1, E2, E3, H1, and H2 can be well assigned to Sb-interstitial (Sb i ), S-vacancy (V S ), Sb S antisite, Sb-vacancy (V Sb ), and S Sb antisite defects, respectively. In the first place, the S deficit in Sb-rich Sb 2 S 3 results in the increase of V S . Excess Sb will then preferentially fill the V S , rather than enter into the interstitial site, since the formation energy of Sb S is essentially lower than that of Sb i . Therefore, the defects V S and Sb S are predominantly appeared in Sb-rich Sb 2 S 3 . However, in S-rich Sb 2 S 3 , S atoms enter lattice to fill the V S initially, and the formations of Sb S and Sb i defects are suppressed due to their increased formation energy in S-rich condition. Afterwards, owing to reduced formation energy, the S-rich condition induces the formation of large amount of V Sb . Furthermore, some S atoms may even occupy the V Sb to form the S Sb antisite in order to maintain the structural stability. Notably, there are only maximum three types of defects detected by DLTS in each Sb 2 S 3 film, much less than those predicted in the theoretical calculations [8] . Fundamentally, the difference between theoretical calculations and experimental measurement can be ascribed to the following two aspects. Firstly, theoretical calculations take all possible defect types into consideration, whereas some of the defects with high formation energy are instable and thus cannot be identified in the measurement. Secondly, DLTS is a technique to detect defects by injecting carriers into depletion region to fill the traps in bulk semiconductors [19] . Accordingly, it is an effective means to probe the deep-level defects in depletion region, especial for which cannot be activated or ionized at room temperature, whereas it is not sensitive to shallow-level defects or defects at interface. These two features result in less defect detected when compared with the theoretical study. In line with the energy level alignment (Fig. 5a, b ), these are all deep-level defects whose energy level is more than 0.3 eV far from CBM or VBM. Therefore, they act as carrier traps or recombination sites due to their high ionization energy. Specially, the trap E2, E3, H1, and H2 feature on deeper energy level (close to intrinsic E F ), large capture cross section and high trap density (Table 1 ) which accords with basic characteristics of trap-assisted SRH recombination center. Thus, they behave as serious recombination centers to hinder carrier transport and shorten the carrier lifetime. Although the above Raman and XPS characterizations do not show impurities such as antimony oxides in the as-prepared Sb 2 S 3 films, we could not exclude the possibility of tiny amount (beyond detection limit) of oxygen doping affecting the defect properties. In this case, we tailor the composition via post-treatment of as-prepared Sb 2 S 3 films with an O 2 /Ar mixed atmosphere at 200 °C for 20–60 min to intentionally introduce oxygen doping (experimental details are provided in the Supplementary note 3 ). Both the secondary ion mass spectroscopy (SIMS) and XPS spectra (Supplementary Fig. 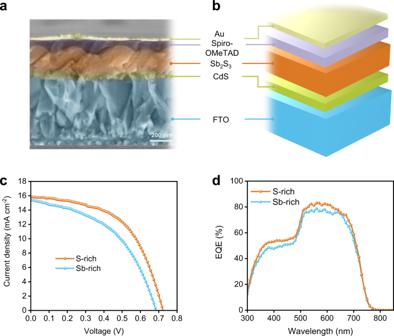5 ) indicate clearly that there is no oxygen existed in as-prepared Sb 2 S 3 films. Fig. 3: Device structure and photovoltaic performance. a,bCross-sectional SEM image and corresponding device configuration of Sb2S3solar cells.cJ–Vcharacteristics of the optimal Sb-rich and S-rich Sb2S3devices under standard one Sun illumination.dEQE spectra of the optimized Sb-rich and S-rich Sb2S3-based devices. After the annealing at 200 °C in O 2 /Ar, the concentration of oxygen is gradually increased from 20 to 60 min (Supplementary Fig. 5c ). We then carry out DLTS analysis. It turns out that oxygen generates remarkable impact on defect properties of Sb 2 S 3 films (Supplementary Fig. 6 , Supplementary Tables 4 and 5 ). In Sb-rich Sb 2 S 3 , the previous three electron traps (E1, E2, E3) are no longer detected, along with the appearance of two hole traps (H1 and H3) after O 2 treatment at 200 °C for 20 min, and even only one hole trap (H3) is observed when the O 2 post-treatment time is prolonged to 40 min. In S-rich Sb 2 S 3 , the previous hole trap H1 is also substituted with another hole trap H3 after O 2 post-treatment, we attribute the trap H3 to O Sb according to defect energy level calculation [8] . Furthermore, the H2 is also passivated when the post-treatment in O 2 was increased to 60 min. On the one hand, we propose that oxygen plays a similar role as sulfur during the processing, which is reasonable since oxygen and sulfur are at the same group in the periodic table. On the other hand, oxygen is more reactive than that of sulfur, it could thus passivate several kinds of defects such as V S , Sb S , and Sb i caused by S deficit, and excessive oxygen would most likely result in the formation of O Sb defects [8] . It is therefore rational that there is finally only one kind of defect like O Sb in the long time (e.g., 60 min) oxygen-treated Sb 2 S 3 films no matter whether the original Sb 2 S 3 is Sb-rich or S-rich (Supplementary Fig. 6 ). According to the above discussion, we can conclude that certain amount of oxygen could induce distinct defect property, particularly in the defect types. Considering that there is no oxygen impurities detected in the as-prepared Sb 2 S 3 films (or negligible amount of oxygen that is beyond detection limit), the defect properties of as-prepared Sb 2 S 3 film in absence of oxygen post-treatment should not be influenced by the possible impurities. Carrier dynamic analysis To study the charge transport kinetics, we perform transient absorption spectroscopy (TAS) measurement of the Sb-rich and S-rich Sb 2 S 3 films deposited on soda-lime glass. We apply glass/Sb 2 S 3 films without any electron or hole extraction layer as sample for this study, which can reflect unambiguously that the exciton relaxes to ground state through charge recombination in films. The TAS is tracked at a time window of 5−5000 ps using 400 nm pulse laser excitation for Sb-rich and S-rich Sb 2 S 3 films (Fig. 6a, b , Supplementary Fig. 7 ). Strikingly, there appear two photo-induced absorption peaks near 545 and 690 nm, both of which are assigned to a single broad feature of trapped carrier in Sb 2 S 3 . Especially, the peak at 690 nm is associated with the formation of sulfide radical [22] , [23] . 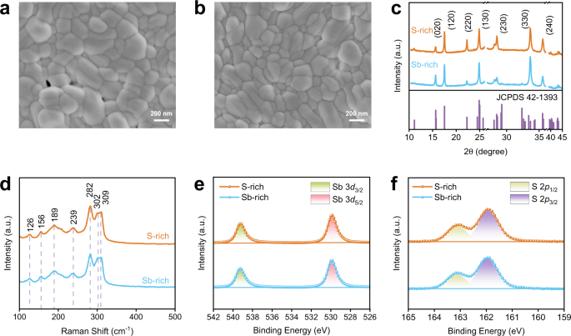Thus, the enhanced absorption at 690 nm for S-rich Sb 2 S 3 could be attributed to abundant sulfide radical. Accordingly, the decay characteristics at 545 nm are fitted by biexponential model to study carrier decay kinetics (Fig. Fig. 2: Characterizations of Sb2S3films. a,bSurface SEM images of Sb-rich and S-rich Sb2S3films.c,dXRD patterns and Raman spectroscopy of Sb-rich and S-rich Sb2S3films.e,fSb 3dand S 2pXPS spectra of Sb-rich and S-rich Sb2S3. 6c and Supplementary Table 2 ). It is observed that the S-rich Sb 2 S 3 exhibits much longer carrier lifetime (18.7 ns) than Sb-rich Sb 2 S 3 (3.8 ns), the reduced defect type and concentration contribute to the prolonged lifetime. Fig. 6: Transient absorption spectroscopy (TAS) study of Sb 2 S 3 films. a , b 2D color images of TAS of Sb-rich and S-rich Sb 2 S 3 films on glass substrates. c Transient kinetic decay (scatter) and fittings according to biexponential decay function (solid lines) monitored at 545 nm of Sb-rich and S-rich films. Δ A is defined as variation of absorption. Full size image To gain further insight into the specific influence of each defect on the carrier dynamics, we extract the limited carrier lifetime associated with specific defect by trap-assisted SRH recombination according to Eq. 1 . τ =(υ_thσN_T)^-1. (1) where the υ th is thermal velocity for electron (hole) that is about 10 7 cm s −1 in bulk semiconductors at room temperature [2] , [3] , [24] . Both σ and N T can be obtained from DLTS. Consequently, the defect with large capture cross section, high density and deep energy level are much more detrimental to carrier lifetime. In Sb-rich Sb 2 S 3 film, the carrier lifetime is limited by trap E2 (V S ) and E3 (Sb S ) in Sb-rich Sb 2 S 3 film which are estimated to be 64.6 and 28.4 ns (Table 1 ), respectively. The other defect E1 (Sb i ) present carrier lifetime of 2180 ns, much longer than those of E2 and E3. This result should be associated with the crystal structure where the Sb atoms entering into the space between (Sb 4 S 6 ) n ribbons is less detrimental to the carrier transport dynamics. In S-rich Sb 2 S 3 film, the trap H1 (V Sb ) sets the limited lifetime of 48.3 ns, while the lifetime limited by trap H2 (S Sb ) is 997 ns. Defect S Sb shows less detrimental to carrier lifetime since the lower concentration due to higher formation energy [9] , even though it manifests deeper energy level than V Sb . We further compare the shortest carrier lifetime limited by E3 and H1, we suppose that this prolonged carrier lifetime is attributed to reduced capture cross section and trap density of H1. In fact, the recombination form in real semiconductors is mainly multi-level recombination [24] . That is to say, the carriers leap among multiple trap level and get recombination ultimately. Therefore, the decreased defect numbers in S-rich Sb 2 S 3 also contribute the longer carrier lifetime. It is worth noting that the calculated carrier lifetime estimated based on bulk trap-assisted SRH recombination model should be slightly exaggerated since it does not consider other non-radiation recombination such as Auger recombination and interface recombination. In any case, the carrier lifetime calculated by bulk trap-assisted SRH recombination model shows the similar trend at the same scale when compared with that obtained by TAS, suggesting that it is the intrinsic deep-level defect that restricts the carrier lifetime in Sb 2 S 3 . For the Sb 2 S 3 solar cell development, one of the major concerns is the efficiency improvement. The rational engineering of the defect properties benefits the carrier transport and suppressing the negative recombination, which further improve three device parameters, V OC , J SC , and FF. In particular, it has been acknowledged that there is a serious V OC loss in the Sb 2 S 3 solar cell. Fundamentally, the V OC of solar cell originates from the split of quasi-Fermi level of electron and hole (Fig. 5c ) [24] , [25] . The trap E2 and E3 in Sb-rich Sb 2 S 3 films with large capture cross section and high trap density, especially trap energy level closer to Fermi level compared with H1 and H2 in S-rich Sb 2 S 3 . There is high possibility that the electron quasi-Fermi level is pinned near trap E2 and E3 in Sb-rich Sb 2 S 3 owing to inefficient extraction of trapped photo-exited carriers. In contrast, S-rich Sb 2 S 3 displays decrescent capture cross section, defects density and defects numbers which jointly give rise to suppressed recombination and prolonged carrier lifetime. This characteristic is able to alleviate the Fermi level pinning effects and improving V OC ultimately. An interesting finding in this study is that the existence of Sb i in the Sb-rich Sb 2 S 3 film generates less detrimental effect on the carrier lifetime, which should be related to Q1D crystal structure where the space between (Sb 4 S 6 ) n ribbons can afford impurities to certain degree. However, the S i defect does not appear in the S-rich Sb 2 S 3 film, it is most likely that the sulfur is easy to be evaporated out during the film deposition at high temperature. Finally, we find that the Sb-rich film displays two types of crucial defects, i.e., V S and Sb S , while S-rich Sb 2 S 3 film shows only one kind of critical defect, V Sb . Therefore, the S-rich Sb 2 S 3 film seems more promising for achieving next efficiency breakthrough, provided that the V Sb is well suppressed without introducing other deep-level defects. Preparation of Sb 2 S 3 thin films The Sb 2 S 3 films were deposited on FTO/CdS substrate preheated at 300 °C via thermal evaporation under pressure of 0.2–0.3 Pa. About 0.3 g Sb 2 S 3 powder (99.9%, aladdin) was put into a tungsten boat equipped on the DC evaporator source, and the evaporating temperature was tuned through the DC current. As for co-evaporation, another 0.1 g S powder (99.999%, Sinopharm group) was needed to evaporate simultaneously with Sb 2 S 3 powder. The films were deposited at a rate of 3–5 nm s −1 . The final thickness of films was controlled around 200 nm via a film thickness gauge. Finally, the as-deposited films were post-annealed at 350 °C for 2 min on a preheated hot plate in a N 2 -filled glove box. Fabrication of Sb 2 S 3 solar cells The FTO glass (TEC-A7) was cleaned by DI water, isopropanol, acetone, and ethanol sequentially. Then FTO substrate was cleaned for 15 min by UV ozone prior to use as well. Next, the FTO substrate coated with 60 nm CdS film as ETL by using chemical bath deposition (CBD) method [4] . After treatment with CdCl 2 (20 mg mL −1 methanol), then FTO/CdS substrate was heated at 400 °C for 10 min in open air. Subsequently, the Sb 2 S 3 film was deposited on FTO/CdS substrate by thermal evaporation mentioned above. Spiro-OMeTAD (Advanced Election Technology Co., Ltd.) was utilized as HTL according our pervious report [5] . Finally, the Au back electrode was evaporated on the HTL under a pressure of 5 × 10 −4 Pa. The active area was defined as 0.12 cm −2 by mask. Film characterizations The morphologies of Sb 2 S 3 thin films were characterized by Zeiss G450 SEM equipped with an EDS (Bruker) module. The crystal structure was measured by XRD (Bruker Advance D8 diffractometer) with Cu Kα radiation ( λ = 1.5406 Å). Raman spectroscopy (Horiba JobinYvon, LabRAM HR800) was applied to analyze chemical bonds of the films with 532 nm laser excitation. XPS (Thermo Fisher) with a Monochrome Al Kα (1486.6 eV, 15 kV) was used to characterize the surface composition. The work function and valence band binding energy were measured by UPS (Thermo Escalab 250Xi, He I excitation 21.22 eV) which were recorded at 0 V samples bias in an ultrahigh vacuum chamber. Secondary ion mass spectroscopy was performed by TOF.SIMS (IONTOF, Germany). TAS of Sb 2 S 3 films were measured by a Helios setup, where a nondegenerate pump–probe configuration was applied to probe the transient dynamics (50 fs to 7 ns). Additionally, the pump and probe laser pulses were generated by frequency doubling the fundamental output (Coherent Vitesse, 80 MHz, Ti-sapphire laser) and white light generated with a sapphire plate, respectively. The decay characteristics were fitted by biexponential model y = Σ A i exp(− x / t i ), while carrier lifetime ( τ ) was obtained by τ = Σ A i t i 2 /Σ A i t i ( i = 2). Device characterizations The J–V characteristics were performed by Keithley 2400 apparatus under solar-simulated AM 1.5 sunlight (100 mW cm −2 ) with a standard xenon-lamp-based solar simulator (Oriel Sol 3 A, Japan). Prior to test, the solar simulator illumination intensity was calibrated by a monocrystalline silicon reference cell (Oriel P/N 91150 V, with KG-5 visible color filter) which is also calibrated by the National Renewable Energy Laboratory (NREL). The EQE (model SPIEQ200) was measured using a single-source illumination system (halogen lamp) combined with a monochromator. The DLTS measurement was performed via a Phystech FT-1230 HERA-DLTS system equipped with a 10-mW red (635 nm wavelength) laser. The optical pulse was generated from the laser via systematical program control. The modified Boonton 7200 capacitance meter (1–75 kHz) was used to examine dynamic capacitance. An n–i–p structural device was selected as one sample, and the effective test area is about 0.01 cm −2 . 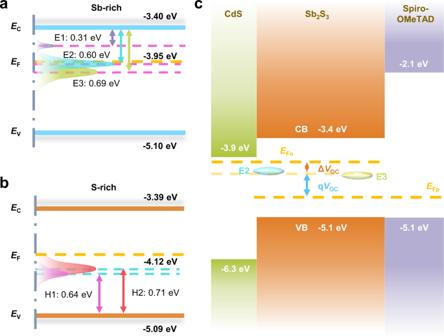Fig. 5: Schematic of band structure and heterojunction. a,bConduction band (EC), valence band (EV), Fermi level (EF), and trap energy level (ET) for Sb-rich and S-rich Sb2S3films.cSchematic diagram ofVOCderived from split of electron and hole quasi Fermi level (EFnandEFp). 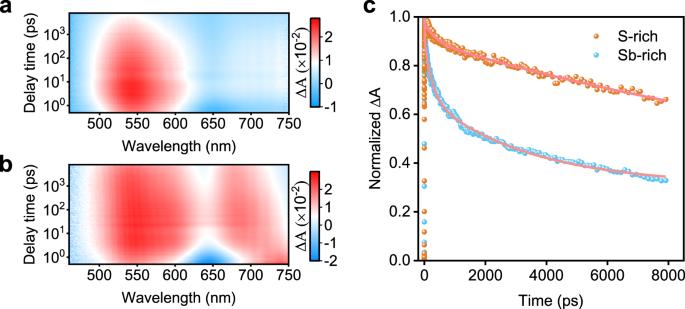Fig. 6: Transient absorption spectroscopy (TAS) study of Sb2S3films. a,b2D color images of TAS of Sb-rich and S-rich Sb2S3films on glass substrates.cTransient kinetic decay (scatter) and fittings according to biexponential decay function (solid lines) monitored at 545 nm of Sb-rich and S-rich films. ΔAis defined as variation of absorption. Then the samples were placed in a liquid-helium cryostat (Lakeshore 335,336). The DLTS temperature scan range was from 120 to 420 K at 2 K heating intervals. The pulse mode was set as electrical (pulse voltage) and optical (laser excitation) double pulse, and they were exerted and removed simultaneously. In detail, the reverse bias, pulse voltage, pulse width (electric and optical), and period width were −0.3 V, 0.1–0.5 V, 10 ms, and 100 ms, respectively. Reporting summary Further information on experimental design is available in the Nature Research Reporting Summary linked to this paper.